Acoustic cavities in 2D heterostructures Two-dimensional (2D) materials offer unique opportunities in engineering the ultrafast spatiotemporal response of composite nanomechanical structures. In this work, we report on high frequency, high quality factor ( Q ) 2D acoustic cavities operating in the 50–600 GHz frequency ( f ) range with f × Q up to 1 × 10 14 . Monolayer steps and material interfaces expand cavity functionality, as demonstrated by building adjacent cavities that are isolated or strongly-coupled, as well as a frequency comb generator in MoS 2 /h-BN systems. Energy dissipation measurements in 2D cavities are compared with attenuation derived from phonon-phonon scattering rates calculated using a fully microscopic ab initio approach. Phonon lifetime calculations extended to low frequencies (<1 THz) and combined with sound propagation analysis in ultrathin plates provide a framework for designing acoustic cavities that approach their fundamental performance limit. These results provide a pathway for developing platforms employing phonon-based signal processing and for exploring the quantum nature of phonons. Acoustic cavities capable of providing spatial confinement for high frequency (1–10 GHz) elastic waves embody a vital part of optomechanical signal processing [1] , [2] , [3] , [4] , [5] , [6] . The ongoing search for implementations of high quality factor ( Q ) acoustic cavities operating in the extremely high frequency range (EHF, 30–300 GHz) is strongly motivated by the promise that nanomechanical devices invoking quantum behavior [1] , [2] , [7] , [8] will allow for an extended temperature range suitable for reaching zero-point motion. Coupling EHF mechanical strain to an embedded nanoscale quantum system (e.g., quantum emitter) [9] , [10] , [11] is another area where the extended frequency range may enable devices suitable for interfacing phonons with two-level systems. However, the low phonon speed that is advantageous for 1–10 GHz devices [3] (and is much celebrated for enabling small device footprints), becomes a challenge as the operational frequency exceeds ~100 GHz. In this frequency regime, the longitudinal phonon wavelength enters the nanometer size range and the critical dimensions fall beyond the limits of electron-beam-based microfabrication methods, thus necessitating a different approach in cavity design. Two-dimensional (2D) materials enable the fabrication of single-crystal, suspended mechanical structures as thin as a single monolayer and represent a promising platform for confining EHF longitudinal acoustic (LA) phonons where free surfaces are utilized as acoustic mirrors. The ultrafast mechanical response of transition metal dichalcogenide (TMD) films was shown to include coherent LA phonons in the frequency range extending up to 1 THz [12] , [13] , [14] , [15] as the film thicknesses decrease to a few monolayers. The mismatch in acoustic impedance between clamped exfoliated layers and their underlying substrate allow for trapping of optically-generated elastic waves with quality factors on the order of Q ≈5 at frequencies up to 200 GHz [12] , [14] , [15] . Significantly longer lifetimes for LA phonons (τ ph = 0.36 ns at 100 GHz) were reported for suspended MoSe 2 films where radiative acoustic losses were excluded [13] . The corresponding improvement in quality factor (Q MoSe2 at 100GHz ≈ 100) puts 2D material-based cavities on a par with implementations based on acoustic distributed Bragg reflectors (DBR) grown by molecular beam epitaxy (MBE) in systems like GaAs/AlGaAs [16] , [17] , [18] . A drastic reduction in cavity modal volume intrinsic to suspended 2D devices represents a significant advantage over DBR cavity implementations, where limited acoustic contrast attainable for MBE-compatible materials (e.g., Z GaAs /Z AlAs = 1.2) causes the elastic strain to extend over 10–20 acoustic wavelengths, even for fine-tuned DBRs (e.g., ref. [19] ). In view of these developments, the fundamental factors that define the highest Q -values attainable in 2D-based acoustic cavities become of prime importance, as well as the prospects of engineering the ultrafast mechanical response of composite 2D devices in order to extend acoustic cavity functionality. In this work, we present an experimental study and theoretical analysis of LA phonon lifetimes in MoS 2 and h-BN that are chosen as an exemplary set of 2D materials with distinct optomechanical properties. We demonstrate that at room temperature (RT), LA phonon lifetimes attainable in MoS 2 -based EHF acoustic cavities (τ MoS2 ≈ 2 ns at 100 GHz, Q ≈ 600) are the highest reported to date for 2D materials and provide a comparison with h-BN based cavities (τ hBN ≈ 0.2 ns). The high spectral purity of MoS 2 devices allows us to study the effects of a unique structural feature for layered materials —monolayer steps—introduced in cavities as a functionality-enabling heterogeneity. We demonstrate laterally-abutted, step-detuned 2D acoustic cavities that behave independently, while being simultaneously accessible for optical excitation and readout. In compound laminar structures, where the heterogeneity is implemented as a MoS 2 /h-BN interface, we exploit cross-plane strain patterns to build a frequency comb generator with nine overtones in the frequency range extending up to 300 GHz. This concept is further extended to a tri-layer MoS 2 /h-BN/MoS 2 structure, where we show that the acoustic spectrum of the laminar structure is related to vibrational modes of two vertically stacked MoS 2 cavities coupled through a more compliant thin h-BN layer. An estimate for the coupling strength of Γ = 47 GHz greatly exceeds the linewidth of the cavity and indicates strong coupling, which offers opportunities in phonon-based signal processing. Finally, the anharmonicity-limited acoustic phonon lifetimes in these systems are evaluated using first-principles density functional theory (DFT) calculations. Given the highly anisotropic nature of 2D materials and the fact that the period of mechanical vibrations of interest is commensurate with the lifetimes of thermal phonons at RT (ωτ th ≈ 1), our atomistic approach provides higher confidence in assessing the fundamental loss contributions in these systems. We use quantum perturbation theory, i.e., Fermi’s golden rule, to determine phonon–phonon scattering rates in which the phonon dispersions and the scattering interactions between phonons are obtained from DFT. These calculations highlight the difference in EHF LA phonon lifetimes between MoS 2 and h-BN and are in good agreement with measurements, indicating that the performance of RT 2D acoustic cavities in the 100–200 GHz frequency range approaches the fundamental limit. Experimental approach The acoustic structures examined here were assembled using a rapidly developing set of fabrication tools [20] , [21] , [22] that enable the formation of 2D laminates with material quality comparable to MBE films, while alleviating the restrictions intrinsic to MBE (e.g., lattice matching, thermal expansion). MoS 2 and MoS 2 /h-BN structures were prepared using either one-step direct mechanical exfoliation or sequential stamping and transfer of flakes onto gold-coated substrates with pre-etched wells (see Fig. 1a , METHODS, and Supplementary Figs. 1 , 2 ). Fig. 1: Mechanical response of acoustic cavities implemented as suspended 2D films. a Schematic showing MoS 2 and MoS 2 /h-BN films on a Ti/Au-coated substrate with pre-etched circular wells. b Snapshot of the normalized ε ZZ mechanical strain (color coded) in the vibrating part of the MoS 2 suspended plate as predicted by time-dependent FEM analysis. The pump beam is modeled as Gaussian with radius 0.5 μm. The part of the plate included in the model is limited by the radius 2 μm with low-reflecting outer boundaries. c Time-dependent reflectivity of a suspended MoS 2 film, shown for delay time between 0.15 and 0.9 ns in parts per million (ppm). d Examples of normalized FFT spectra of the time-dependent reflectivity taken from different MoS 2 cavities. The high frequency peaks are labeled with the corresponding MoS 2 film thicknesses in layer number as extracted from Raman spectroscopy data (see frequency vs. layer number dependence in Supplementary Fig. 2 ). The peaks are displayed in different colors to help readability. e Frequency versus layer number for a range of MoS 2 acoustic cavities. (inset) f × Q of MoS 2 cavities as a function of frequency. The dashed line shows the value required for ground state cooling (6 × 10 12 Hz). The red curve is added as a guide-to-the-eye and was obtained as a fit using a logistic distribution. Variability in f × Q values for different cavities in the vicinity of 150 GHz is illustrated by the blue star points with f × Q average = 0.7 × 10 14 . Full size image An ultrafast near infrared (NIR) optical pump-probe setup with spatial resolution of about 1 μm was used to evaluate the local, time-resolved mechanical response of the suspended structures. We refer to the portions of the 2D structures undergoing optically-generated thickness-mode vibrations as “acoustic cavities,” and consider these as an extension of the trapped energy resonator concept [23] . Given the semiconducting nature of MoS 2 , the deformation potential is likely to be the dominant mechanism for generating optically-induced elastic strain [24] , [25] . The large penetration depth for the pump laser (770 nm) in MoS 2 ensures uniform excitation and thus homogeneous initial stress along the normal component. Optical readout for the mechanical response is provided by delayed probe pulse (830 nm wavelength), as its reflectivity is modulated by both film dilation (Fig. 1b ) and photoelastic effects [26] , [27] , also magnified by interferometric effects via a Fabry–Perot optical cavity (see METHODS). Finite element modeling (FEM) [28] was used to analyze and to interpret the outcome of pump-probe experiments. Calculations fully account for the anisotropy of bulk TMD materials and h-BN. In accord with Greener et al. [15] , continuum elasticity-based models were consistent with the experimental results in the sub-THz frequency range. MoS 2 acoustic cavities The normalized reflectivity (ΔR/R) of a suspended MoS 2 film, after subtracting a slowly varying background, is shown in Fig. 1c as a function of delay time between the pump and probe laser pulses (raw data is shown in Supplementary Fig. 3 ). A pronounced modulation is attributed to the thickness-mode vibrations since the single peak in the FFT spectrum (e.g., Fig. 1d ) matches the expected resonance frequency for a sound wave where a half-wavelength fits across the film thickness (146.25 GHz for the 18-layer (18 L), 11.2 nm film in Fig. 1c ). The variation of the FFT spectra with the film thickness measured in number of monolayers N (0.62 nm per layer for MoS 2 [29] ) is shown in Fig. 1e and follows the expected trend of f ∼ N −1 (see for example ref. [13] ). Fitting the data in Fig. 1e provides an average value for the cross-plane LA sound speed c LA = 3170 m/s in our MoS 2 films. The slow decay of the pump-induced vibrations (Fig. 1c ) indicates minimal energy losses and highlights a low internal friction of crystalline MoS 2 , as well as negligible “phonon leaking” (caused by lateral spreading of pump-driven elastic excitations) in the 100 GHz-range TMD cavities. A ring-down time of τ ≈ 1.6 ns that is extracted via fitting an exponentially-decaying time dependence to the vibrational amplitude in Fig. 1c corresponds to a cavity quality factor Q = 730 at f = 146.25 GHz. For this cavity, the resulting f × Q = 1.1 × 10 14 Hz is the highest measured in our experiments and also the highest reported to date for a 2D material system (to our knowledge). The physical mechanisms that define the fundamental limits attainable for Q values (i.e., phonon lifetimes) in different 2D materials will be discussed below. While differences in the performance of individual cavities can be 5× (attributed to variability in manual exfoliation), the f × Q product for our MoS 2 devices remains at or above that required for ground state laser cooling ( f × Q = 6 × 10 12 Hz) [30] . 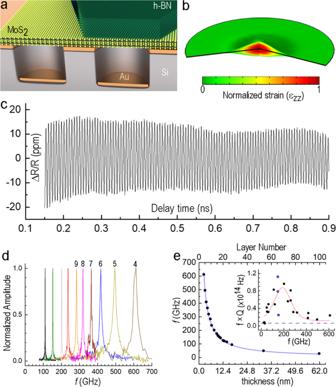Fig. 1: Mechanical response of acoustic cavities implemented as suspended 2D films. aSchematic showing MoS2and MoS2/h-BN films on a Ti/Au-coated substrate with pre-etched circular wells.bSnapshot of the normalized εZZmechanical strain (color coded) in the vibrating part of the MoS2suspended plate as predicted by time-dependent FEM analysis. The pump beam is modeled as Gaussian with radius 0.5 μm. The part of the plate included in the model is limited by the radius 2 μm with low-reflecting outer boundaries.cTime-dependent reflectivity of a suspended MoS2film, shown for delay time between 0.15 and 0.9 ns in parts per million (ppm).dExamples of normalized FFT spectra of the time-dependent reflectivity taken from different MoS2cavities. The high frequency peaks are labeled with the corresponding MoS2film thicknesses in layer number as extracted from Raman spectroscopy data (see frequency vs. layer number dependence in Supplementary Fig.2). The peaks are displayed in different colors to help readability.eFrequency versus layer number for a range of MoS2acoustic cavities. (inset)f×Qof MoS2cavities as a function of frequency. The dashed line shows the value required for ground state cooling (6 × 1012Hz). The red curve is added as a guide-to-the-eye and was obtained as a fit using a logistic distribution. Variability inf×Qvalues for different cavities in the vicinity of 150 GHz is illustrated by the blue star points withf×Qaverage= 0.7 × 1014. Figure 1d, e inset highlight the frequency dependence of energy losses and suggest that the 100–200 GHz frequency range is favorable for maximizing the f × Q product in this measurement geometry at RT. Therefore, we focus on the corresponding range in film layer number, centered at about 10 nm ( N ~16 layers), and demonstrate that the layered nature of 2D materials enables introduction of well-controlled heterogeneities that can alter the underlying elastic-strain patterns and expand cavity functionality by modifying the ultrafast mechanical response. Step-detuned cavities in MoS 2 Toward the goal of employing heterogeneities as acoustic tools, we consider discrete thickness variations, or steps, between atomically-flat regions on a 2D material surface as a reproducible and well-controlled feature for altering the ultrafast response. The high Q value of our MoS 2 cavities allows us to resolve perturbations in the mechanical response of 100 GHz devices induced by the presence of even a single monolayer step. 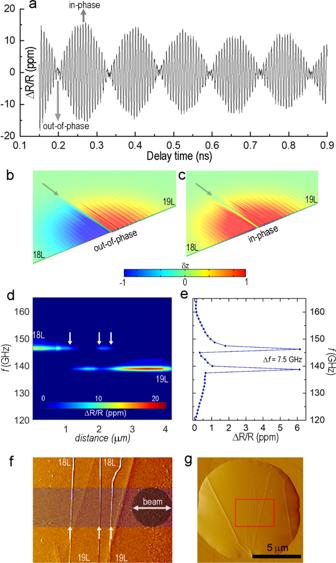Fig. 2: Horizontally-abutted cavities divided and detuned by a monolayer step. aTime-dependent reflectivity taken at a monolayer step boundary on an 18-layer (18 L)/19-layer (19 L) MoS2suspended film. The in-phase and out-of-phase labels show the timing for the snap-shots inb,c. FEM-generated snapshots of normalized vertical displacement maps (δz) highlighting the out-of-phase (b) and in-phase (c) vibrations of the abutted cavities at the monolayer step. Additional information for the time-domain FEM analysis are included in the Supplementary Information (Supplementary Note2and Supplementary Movie1).d2D plot showing color-coded FFT spectra of the probe reflectivity acquired at different positions while stepping the beam across the monolayer steps shown inf.eFFT spectrum of time-dependent reflectivity froma, which is taken approximately at the 2.2 μm position ind.fAFM phase-image showing the region where the spectra inaanddwere acquired. The monolayer steps run vertically across the image. The horizontal darkened band shows the path where the 1 μm diameter beam was scanned across the surface.gLow magnification AFM phase-image showing the MoS2drum (see Supplementary Fig.4for optical image). The red box highlights the region imaged inf. Figure 2a shows the time-dependent reflectivity acquired for a suspended MoS 2 film with a 1 L step positioned at the center of the coinciding pump/probe beams (optical image in Supplementary Fig. 4 ). Fig. 2: Horizontally-abutted cavities divided and detuned by a monolayer step. a Time-dependent reflectivity taken at a monolayer step boundary on an 18-layer (18 L)/19-layer (19 L) MoS 2 suspended film. The in-phase and out-of-phase labels show the timing for the snap-shots in b , c . FEM-generated snapshots of normalized vertical displacement maps (δz) highlighting the out-of-phase ( b ) and in-phase ( c ) vibrations of the abutted cavities at the monolayer step. Additional information for the time-domain FEM analysis are included in the Supplementary Information (Supplementary Note 2 and Supplementary Movie 1 ). d 2D plot showing color-coded FFT spectra of the probe reflectivity acquired at different positions while stepping the beam across the monolayer steps shown in f . e FFT spectrum of time-dependent reflectivity from a , which is taken approximately at the 2.2 μm position in d . f AFM phase-image showing the region where the spectra in a and d were acquired. The monolayer steps run vertically across the image. The horizontal darkened band shows the path where the 1 μm diameter beam was scanned across the surface. g Low magnification AFM phase-image showing the MoS 2 drum (see Supplementary Fig. 4 for optical image). The red box highlights the region imaged in f . Full size image Pronounced beats observed during the ring-down (Fig. 2a ) manifest as two distinct peaks in the FFT spectrum (see below), in striking contrast to the monochromatic response of homogeneous cavities in Fig. 1d . The split Δf ≈ 7.5 GHz between the experimentally observed peaks in the spectrum of the “step-cavity” closely matches the detuning expected from a monolayer change in thickness and suggests that the excited parts of the film on each side of the step behave as co-vibrating, but nearly isolated acoustic cavities. Such interpretation implies that the experimentally observed beats in the intensity of the reflected probe pulse arise when the photodetector sums up the contributions from two concurrent but frequency-shifted vibrational modes (Fig. 2b, c ). If we assume that some degree of coupling is present between the half-cavities, these vibrational modes could be considered as mixed modes (ω ± ) of coupled resonators (see for example ref. [31] and Supplementary Note 1 ). In the weak coupling limit κ coupling → 0, the frequencies of the mixed modes are expected to approach those corresponding to flat plates (18 L and 19 L). To evaluate the coupling strength, we compare the vibrational spectra acquired on the step with the response far away from the step. Figure 2d shows a filled contour plot of the spatially varying FFT spectra (see example of a single spectra in Fig. 2e ) as coinciding pump/probe beams are moved laterally across the monolayer steps imaged in Fig. 2f, g . Regardless of the measurement position (“on step” or “away from step”) we only observe a set of discrete frequencies, each corresponding to a whole number of MoS 2 monolayers. There is no evidence of frequency deviation for the mixed modes in the vicinity of the steps, at least not within the signal-to-noise ratio available in our experiments. This result indicates that despite the cavities being formed mostly by the same atomic planes, the lateral coupling between the abutted cavities does not exceed the halfwidth of the resonance (≈0.2 GHz). Employing a one degree-of-freedom (1DOF) model for two coupled and nearly identical oscillators [31] (Supplementary Equation 3 ), this result provides an upper boundary estimate for the spring constant ratio κ coupling /k oscillator ≈ 2 × 10 −3 , implying nearly independent cavities. This estimate confirms that in contrast to “acoustic molecules” [32] , the energy transfer between laterally abutted 2D cavities is negligible, at least within the pump repetition period in our experiments. Therefore, the low frequency envelope in Fig. 2a provides the frequency difference between the abutted half-cavities (ω + –ω − , Fig. 2a ), where each can be viewed as independent. We emphasize that such a differential readout is enabled by the nature of well-defined monolayer steps in 2D materials and note that recently developed transfer methods allow for controlled placement of such steps in top-down lithographical approaches (e.g., adding a monolayer film on half of a uniformly thick slab [33] ). Simultaneous optical response from the adjacent acoustic cavities can enable frequency down-conversion, where one of the half-cavities acts as a local oscillator for the other half-cavity. Recent progress in developing nonlinear optical detectors [34] opens the possibility for mixing intensity-modulated optical signals coming from the abutted-cavities directly at the photodetector. An estimated bandwidth of ~0.5 THz for the graphene-based mixer-detector [34] could allow real-time down-conversion with the output electric signal from the photodetector modulated at the beat frequency of adjoined TMD cavities. We also note that although our experiments do not show cyclic energy exchange between the half-cavities, a step on the area of the plate that undergoes thickness-mode vibrations can generate a steady energy outflow (i.e., leakage) by launching slow propagating longitudinal elastic waves known as Lamb waves [23] , [35] . These waves are manifested as the ripples seen in Fig. 2b, c and for a nanostructure embedded in the plate, they can make a remote, high- Q , pulse-driven step-cavity to appear as a narrow-band Lamb wave generator with the frequency defined by the plate thickness. While beyond the scope of this work, this concept can open opportunities for in-plane (“on-chip”) EHF acoustics. Unfortunately, within our experimental approach, these effects are muted by the disparity between the lateral extent of the diffraction-limited probe laser spot and the much shorter in-plane wavelengths of step-generated elastic excitations. h-BN/MoS 2 bilayer: Frequency comb and h-BN phonon lifetime To provide stronger coupling for our optical readout system, we explore heterogeneities that span the full laser spot diameter, such as those formed at the boundaries of dissimilar materials in laminar structures. Modifications to an acoustic cavity that enable access to high-frequency overtones can be implemented by invoking highly nonuniform strain patterns for the cavity excitation. To ensure such a nonuniformity in a laminated stack of 2D materials, we assembled devices composed of a relatively thick h-BN layer (44 nm) van der Waals (vdW) bonded to a thinner MoS 2 layer (8.7 nm or 14 L; optical image in Supplementary Fig. 4 ). The large disparity in material bandgaps (h-BN ≈ 6 eV and bulk MoS 2 ≈ 1.2 eV) limits optical absorption of the pump beam to the MoS 2 layer alone, thereby making the TMD a thin transducer that drives the full 53 nm thick stack. 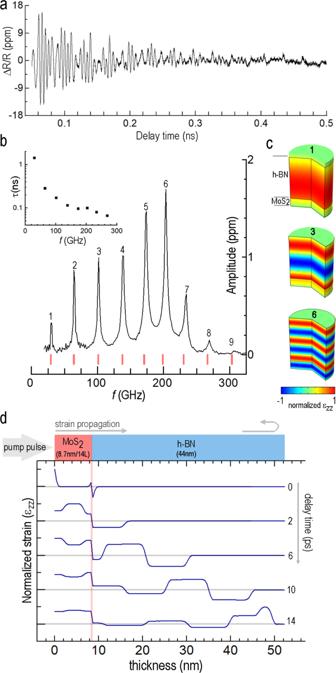Fig. 3: Frequency comb generator implemented in a h-BN/MoS2bilayer. aTime-dependent reflectivity for a h-BN (44 nm)/MoS2(8.7 nm/14 L) suspended film.bFFT spectrum of the signal shown ina. The red tick marks along the bottom of the plot show positions of the bilayer overtones as predicted by FEM eigenfrequency analysis. The peaks are numerically labeled from lowest to highest frequency. (inset) Extracted lifetimes for h-BN (τhBN) versus frequency for peaks inb(see Supplementary Note4for details of the extraction method).cSpatial configuration of the normalized εZZstrain for three different modes (labeled) in the h-BN/MoS2heterostructure (eigenfrequency FEM analysis, 1D model).dSnapshots of the εZZstrain distribution generated by optically-excited MoS2are shown across the thickness of the bilayer at early delay times (for details of time-domain axisymmetric FEM analysis, see Supplementary Note3). Figure 3a shows the time-dependent reflectivity from a h-BN/MoS 2 heterostructure, which is notably different from both the homogenous cavities in Fig. 1 and the “step-cavities” in Fig. 2 . Despite the complex appearance, the temporal behavior is straightforward to interpret in the frequency domain, where a pronounced frequency comb emerges with a series of nearly equidistant peaks with separation Δ f ≈ 34 GHz (Fig. 3b ). Using eigenfrequency numerical analysis, we find that the center frequency for each experimentally observed peak coincides with that of corresponding high-order overtones (red ticks) in the laminated h-BN/MoS 2 structure. Examples of the spatial configuration of the strain for the high-order overtones can be seen in Fig. 3c . The frequency comb extends to the ninth-order overtone and spans nearly four octaves, which is unattainable for a uniformly excited homogeneous film (e.g., Fig. 1d ). The larger amplitudes of high-order overtones in Fig. 3b are directly related to the highly inhomogeneous strain generated across the h-BN/MoS 2 stack by the pump pulse. Figure 3d shows snapshots of strain patterns calculated using time-domain FEM analysis (see Supplementary Note 3 for details of the modeling approach). Expansion of the MoS 2 film is driven by the deformation potential [25] and generates a succession of nearly rectangular strain pulses launched into the h-BN layer, which then propagate at the speed of the longitudinal sound waves ( c LA ≈ 3.4 × 10 3 m/s for h-BN; the snap-shots of the spatial distribution for the out-of-plane strain in the bilayer are shown in Supplementary Figs. 6 , 7 and Supplementary Movie 2 ). The envelope of the comb in the experimentally acquired spectrum (Fig. 3b ) peaks at about 200 GHz and is defined by the sample geometry. An overtone is prominent when the wavelength of the standing wave, λ s (see Fig. 3c ) closely matches that of the elastic wave launched by the MoS 2 transducer in response to pulse excitation (Fig. 3d ). Here, the sixth overtone (~200 GHz, strain pattern in Fig. 3c ) has the closest overlap since the MoS 2 layer thickness approaches the half-wavelength, λ s /2. Accordingly, the inverse round-trip time for sound within the MoS 2 is commensurate with the overtone’s frequency. Fig. 3: Frequency comb generator implemented in a h-BN/MoS 2 bilayer. a Time-dependent reflectivity for a h-BN (44 nm)/MoS 2 (8.7 nm/14 L) suspended film. b FFT spectrum of the signal shown in a . The red tick marks along the bottom of the plot show positions of the bilayer overtones as predicted by FEM eigenfrequency analysis. The peaks are numerically labeled from lowest to highest frequency. (inset) Extracted lifetimes for h-BN ( τ hBN ) versus frequency for peaks in b (see Supplementary Note 4 for details of the extraction method). c Spatial configuration of the normalized ε ZZ strain for three different modes (labeled) in the h-BN/MoS 2 heterostructure (eigenfrequency FEM analysis, 1D model). d Snapshots of the ε ZZ strain distribution generated by optically-excited MoS 2 are shown across the thickness of the bilayer at early delay times (for details of time-domain axisymmetric FEM analysis, see Supplementary Note 3 ). Full size image The bilayer h-BN/MoS 2 geometry used here provides a point of comparison with a similar transduction approach based on spatially-inhomogeneous optical absorption that has been used to generate a broadband frequency comb in GaAs/AlGaAs/InGaAs systems [36] , [37] . A distinct advantage offered by 2D materials is the higher level of spatial confinement, which is illustrated by comparing our 53 nm thick h-BN/MoS 2 stack versus the combined 407 nm thick multiple quantum well structures (plus 3.76 μm for the DBR reflector) in ref. [37] . More importantly, given the wide frequency range of excited overtones, our measurement provides experimental evaluation for the frequency dependence of the longitudinal phonon lifetimes in h-BN (Fig. 3b inset), as the energy dissipation in our bilayer structure can be separated into individual contributions from h-BN and MoS 2 (see for example ref. [38] and Supplementary Note 4 with the elastic energy distribution for different vibrational modes in the bilayer shown in Supplementary Fig. 8 , and energy partitioning coefficients listed in Supplementary Table 1 ). These results are enabled by the high-quality, low-loss MoS 2 transducer layer since h-BN alone would be inaccessible for a NIR wavelength pump-probe setup. While a metal transducer evaporated on a semiconductor film can also be used to generate a frequency comb [39] , [40] , the use of a crystalline 2D material-based transducer with low internal friction and diminished surface roughness can reduce the overall energy losses and make the estimates for the phonon lifetimes more reliable. Importantly, a wide variety of high-contrast bilayer structures with atomically-sharp interfaces can be built using 2D materials. The transfer approach mitigates problems inherent to physical vapor deposition, such as island growth modes (due to dissimilar surface energies) or interdiffusion, as well as built-in stress associated with many evaporated/epitaxial films. Our control experiments with stacked MoS 2 /MoS 2 slabs indicate that the adopted method for flake transfer, including exposure to ambient air does not increase the mechanical losses considerably (see Supplementary Note 5 and frequency dependence of the quality factor Q for MoS 2 /MoS 2 stacks shown in Supplementary Fig. 9 ). Similar low-loss behavior is projected on MoS 2 /h-BN boundaries based on transmission electron microscopy (TEM) results that find pristine interfaces between h-BN and MoS 2 [41] . Close values of interface adhesion energy (0.3 J/m 2 for MoS 2 /h-BN versus 0.4 J/m 2 for MoS 2 /MoS 2 interfaces) also imply commonalities in vdW self-cleansing mechanism for these interfaces [42] and therefore, similar losses. Coupled cavities in MoS 2 /h-BN/MoS 2 tri-layer In the implementation of the frequency comb described above, we centered our analysis on energy dissipation within individual cavity components and on relative intensities of the excited overtones in the bilayer h-BN (44 nm) /MoS 2 (8.7 nm) cavity. Building on this assessment, we extend the multilayer design approach in an effort to reengineer the cavity vibrational modes themselves. To illustrate mode alteration, we sandwich a thin h-BN film between two MoS 2 layers (MoS 2(17L) / h-BN (5L) / MoS 2(15L) ) in an effort to tailor the strain patterns and the corresponding spatial redistribution of the elastic energy across a tri-layer laminar structure (optical images of the tri-layer structures and elastic energy distribution for selected vibrational modes are shown in Supplementary Figs 10, 11 ). 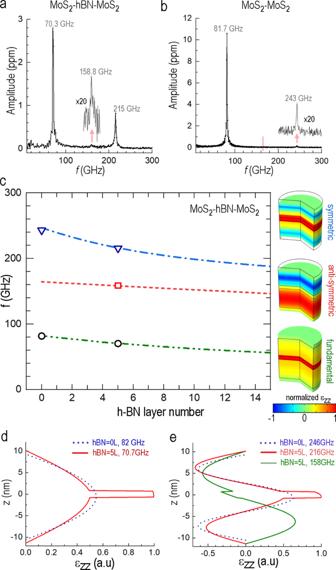Fig. 4: Strongly coupled acoustic cavities constructed as a vertically-stacked heterostructure. aSpectrum for the MoS2/h-BN/MoS2tri-layer;bSpectrum of the neighboring MoS2/MoS2control area. The red tick inbhighlights the location of the non-active second harmonic peak. Only odd modes are excited with the homogeneous pump excitation here.cFEM-predicted frequencies for the three lowest vibrational modes of the tri-layer system as function of the spacer h-BN layer thickness. Experimental data (open symbols) are included for the tri-layer (h-BN thickness = 5 L, normalized εZZstrain configurations are shown on the right) and for the control sample (h-BN thickness = 0 L).d,eThe normalized εZZstrain profiles for vibrational modes in monolithic MoS2(dotted lines) are shown in comparison with strain in the tri-layer system (solid lines) at the labeled frequencies. Figure 4 compares the measured vibrational spectrum for a tri-layer MoS 2(17L) /h-BN (5L) / MoS 2(15L) sample (Fig. 4a ) with the spectrum of a control bi-layer MoS 2(17L) / MoS 2(15L) sample (Fig. 4b ). A significant increase in the intensity of the third overtone (215 GHz, Fig. 4a ) is a notable outcome of introducing the h-BN middle layer. However, even more important is the fact that the position of the second overtone in the tri-layer structure (158 GHz, Fig. 4a ) becomes far detuned from the doubled frequency of the fundamental mode (70.3 GHz). The fundamental mode frequencies for both devices match the FEM-predicted values (Fig. 4c ), which provides confidence that the material interfaces behave as “ideal boundaries” with no softening due to interlayer contamination [15] . Dotted lines in Fig. 4c show the calculated frequencies for the first three vibrational modes of the tri-layer stack as function of the h-BN thickness. The salient feature is the progression from equidistant harmonics in the monolithic MoS 2 film (at h-BN = 0 nm) to a set of second and third overtones (red and blue lines, Fig. 4c ) that converge towards the resonant frequency for an isolated 17L-thick MoS 2 layer (154 GHz). Such a tendency is governed by the strain patterns arising from the presence of the h-BN layer (Fig. 4d, e ). For the second overtone (anti-symmetric, ≈ 158 GHz) the location of h-BN layer coincides with the strain node. As a result, the reduced material stiffness (C 33 = 27 GPa in h-BN [43] versus C 33 = 54 GPa in MoS 2 [44] ) becomes inconsequential in the elastic response. On the contrary, the third overtone (symmetric, 216 GHz) applies maximum strain to the h-BN layer, which leads to a reduced restoring force and lower resonant frequency. The overtones moving closer to each other invoke a model where two MoS 2 slabs can be considered as distinct acoustic cavities coupled through the h-BN barrier. The third overtone is then interpreted as ω + (symmetric) mode, while the second overtone is assigned as ω − mode (see refs. [30] , [31] and Supplementary Notes 1 , 6 ). Experimental data for the overtones’ positions in our tri-layer stack are shown by open symbols in Fig. 4c and demonstrate a clear step toward a coupled-cavity implementation. A 1DOF model for two coupled mechanical oscillators (see Supplementary Equations 3 , 4 ) applied to our tri-layer system produces coupling strength Γ ≈ 47 GHz and κ coupling /k oscillator ≈ 0.35, implying very strong coupling. Fig. 4: Strongly coupled acoustic cavities constructed as a vertically-stacked heterostructure. a Spectrum for the MoS 2 /h-BN/MoS 2 tri-layer; b Spectrum of the neighboring MoS 2 /MoS 2 control area. The red tick in b highlights the location of the non-active second harmonic peak. Only odd modes are excited with the homogeneous pump excitation here. c FEM-predicted frequencies for the three lowest vibrational modes of the tri-layer system as function of the spacer h-BN layer thickness. Experimental data (open symbols) are included for the tri-layer (h-BN thickness = 5 L, normalized ε ZZ strain configurations are shown on the right) and for the control sample (h-BN thickness = 0 L). d , e The normalized ε ZZ strain profiles for vibrational modes in monolithic MoS 2 (dotted lines) are shown in comparison with strain in the tri-layer system (solid lines) at the labeled frequencies. Full size image Apart from the interplay between the high-frequency overtones, the fundamental vibration mode in our tri-layer system is of prime interest since it features a large and nearly uniform strain profile within the h-BN layer (Fig. 4d ). Known to be a good host for RT quantum photon sources [45] , [46] , [47] , [48] , the h-BN spacer layer sandwiched between MoS 2 “hammer and anvil” represents a promising configuration for coupling embedded optical emitters to coherent LA phonons confined in the tri-layer cavity. Importantly, both the maximum attainable strain, as well as the spectral purity of the elastic stimulus delivered to embedded nanostructures are defined by the quality factor of the overall cavity. Energy losses in both the h-BN “device layer” and surrounding MoS 2 structures affect the total phonon lifetime in the cavity. The experimental values for the tri-layer ring-down time τ Total = 0.65 ns fall between our previously extracted values for τ hBN = 0.24 ns and τ MoS2 = 2.8 ns at 70 GHz and agree to within 10% with the prediction 1/τ Total = α 1 /τ hBN + α 2 /τ MoS2 where α 1, α 2 are energy partition coefficients for the tri-layer structure (see Supplementary Table 2 ). We view this agreement as a strong indicator that losses related to the MoS 2 /h-BN interfaces do not limit the phonon lifetime in the cavity. Developing a toolbox for building high-performance acoustic cavities in 2D materials requires a quantitative understanding of the fundamental mechanisms that govern phonon lifetimes, including both frequency and temperature dependences. It is also necessary to account for both material-specific internal friction, as well as extrinsic effects (e.g., surfaces and imperfections, confinement losses, etc.). Intrinsic losses in the nonmetallic materials studied here (at RT) arise mainly from phonon–phonon scattering, often referred to as anharmonic effects. Until recently only semiquantitative models, developed primarily for sound attenuation in isotropic materials and intended for frequency limits ωτ th << 1 or ωτ th >> 1, have been available for fitting measured data (ω is the frequency of the sound wave and τ th is the lifetime of thermal phonons, see for example refs. [49] , [50] ). Advancements in the development of first-principles techniques now allow for fully microscopic treatments of phonon lifetimes [51] , [52] (see Supplementary Notes 7 , 8 for description of theoretical approach), which do not invoke uncertainties resulting from experimentally-derived empirical constants within the model (e.g., average Grüneisen parameters). Relatively little work of this kind has been done in predicting phonon lifetimes for low frequency acoustic phonons [51] , [52] , particularly in comparing with measured data in low dimensional and vdW layered systems. Our calculated phonon lifetimes for all polarizations due to anharmonic three-phonon scattering alone through the Brillouin zones for bulk and monolayer MoS 2 and h-BN are shown in Fig. 5a, b (see METHODS; also see Supplementary Figs. 12 – 14 for schematics of the theoretical setup and Supplementary Figs. 15 , 16 for phonon lifetimes projected onto the phonon dispersion curves, as well as full Brillouin zone data). 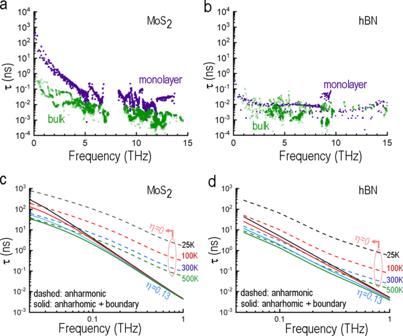Fig. 5: Phonon lifetimes due to anharmonic phonon–phonon scattering for bulk and monolayer systems. Phonon lifetimes through the Brillouin zones for all polarizations and propagation directions at room temperature inaMoS2andbh-BN. For h-BN, phonon lifetimes are truncated at 15 THz. Lifetimes over the entire frequency range are shown in Supplementary Fig.16. Low-frequency plot (log-log) showing temperature dependences of lifetimes for cross-plane LA phonons incMoS2anddh-BN from anharmonic scattering (dashed curves, η = 0) and from the sum of anharmonic scattering and surface losses (solid curves, η = 0.13).ηis the root mean square variation of the surface height (i.e., rms roughness in nanometers). They vary widely in magnitude across each Brillouin zone and become considerably longer at low frequencies. For thermal phonons ( f th = k B T /(2 π ħ ) ≈ 6.25 THz at RT) the predicted lifetime is close to τ th ≈ 1–3 ps for both bulk h-BN and MoS 2 . The ability to cover seamlessly the entire low frequency range ( ħω < k B T ), including the crossover at ω c τ th ≈ 1 (which is of prime interest here at ω c ≥ 2 π × 55 GHz), is a major advantage of our DFT-based approach. The lifetimes in MoS 2 and MoSe 2 (see Supplementary Figs. 15 , 16 ) were found to be similar in overall magnitude, and those in h-BN are somewhat shorter, especially near the f ≈ 1 THz range. To illustrate the versatility of the microscopic approach, we also present the phonon lifetimes calculated for monolayers of MoS 2 , h-BN and MoSe 2 (see Supplementary Fig. 16 ). The enhanced phonon lifetimes predicted for the TMD monolayers MoS 2 and MoSe 2 (though not so for h-BN) suggest that the intrinsic anharmonic losses are less significant in these materials as layer thicknesses are reduced. At lower frequencies in particular, out-of-plane flexure vibrations with quadratic dispersions in monolayer materials tend to have long lifetimes. These modes are not present in their bulk counterparts. Fig. 5: Phonon lifetimes due to anharmonic phonon–phonon scattering for bulk and monolayer systems. Phonon lifetimes through the Brillouin zones for all polarizations and propagation directions at room temperature in a MoS 2 and b h-BN. For h-BN, phonon lifetimes are truncated at 15 THz. Lifetimes over the entire frequency range are shown in Supplementary Fig. 16 . Low-frequency plot (log-log) showing temperature dependences of lifetimes for cross-plane LA phonons in c MoS 2 and d h-BN from anharmonic scattering (dashed curves, η = 0) and from the sum of anharmonic scattering and surface losses (solid curves, η = 0.13). η is the root mean square variation of the surface height (i.e., rms roughness in nanometers). Full size image In order to represent acoustic vibrations in films with varying thicknesses h we use calculations for bulk LA modes polarized perpendicular to the surfaces with wave vectors q z and with half wavelengths equal to the layer thicknesses, h = λ z /2 = π / q z . Their frequencies as functions of thickness are found to agree well with the corresponding measurements in Fig. 1e . The phonon lifetimes due to anharmonic phonon scattering alone in the THz regime for MoS 2 and h-BN are given by the dashed curves in Fig. 5c, d , where they are seen to decrease with frequency. The temperature dependences of the anharmonic contributions to phonon lifetimes for MoS 2 (Fig. 5c ) and h-BN (Fig. 5d ) are pronounced and arise from the phonon population factors in the phonon–phonon scatterings. Lower temperatures can reduce anharmonic scattering losses considerably. To represent the extrinsic contributions to the vibration lifetimes, a simple model for surface losses due to scattering from randomly varying surface or boundary heights [53] is used (solid lines Fig. 5c, d ). This gives a scattering contribution in the form 
    1/τ_surface=1-p/1+p|v_z|/h,p=e^-(4πη/λ_z)^2
 (1) where p is the specularity of the surface, v z is the group velocity, λ z is the acoustic wavelength and η is the root mean square variation of the surface height (i.e., rms roughness). Recent measurements on freshly cleaved MoS 2 surfaces give an estimated η = 0.23 nm [54] , which could be even smaller for clean MoS 2 surfaces with fewer sulfur vacancies and adsorbed species. To assess how well these microscopic calculations compare with our measured data, Fig. 6a shows the experimental ring-down times for the monolithic MoS 2 cavities described earlier (see Fig. 1 ). The sum of the anharmonic and surface roughness losses are in very good agreement with experiment for the frequencies f ≥ 100 GHz, both for magnitude and for frequency dependence. Two different values of η are provided to illustrate the effects of varying surface roughness. The two solid blue curves in Fig. 6a give the sum of these surface losses and the anharmonic scattering for MoS 2 for η = 0.25 nm and for η = 0.13 nm, where the latter is fit to the measured data here (black squares). Fig. 6: Experimental and theoretical results for the lifetimes of LA phonons polarized perpendicular to the basal plane. Frequency dependence predicted for the room temperature phonon lifetimes in a MoS 2 and b h-BN as defined by anharmonic scattering alone (dashed curves; η = 0) and by the combination of anharmonic scattering with surface losses (solid curves; η > 0) for two values of rms surface roughness (η) in nanometers. Values extracted from experimentally measured cavity ring-down times are shown by the black ( a ) and red ( b ) square points. The green points in a and c show the FEM-calculated time for Lamb waves escape LWE (see Supplementary Note 9 for details). c Comparison of calculated and measured f × Q product as a function of frequency. The black lines show f × Q values calculated for MoS 2 cavities and the red lines correspond to h-BN structures at the labeled temperatures and η. Experimental data for cavities studied in the present work are given by the square and star symbols as labeled. The tri-layer data points represent the MoS 2 /h-BN/MoS 2 heterostructure (see Fig. 4 ). Full size image A broad frequency range comparison of our microscopic calculations and experimental data against the well-accepted models for absorption of sound in insulators [55] , based on Landau–Rumer and Akhiezer approach, shows that ab initio predictions for τ in the intermediate range (i.e., ωτ th ≈ 1) are an order of magnitude larger (see Supplementary Fig. 17 for the comparison of ab initio calculations, experimental data, and asymptotic theoretical models). We emphasize that in the absence of the DFT-based results any quantitative analysis of dissipation above 50 GHz (ωτ th ≈1) would be challenging and assumption-driven (see for example ref. [50] ). That frequency range is of prime importance here, since at 100 GHz the performance of our MoS 2 -based cavities is within a factor of three from the fundamental limit defined by the intrinsic anharmonicity-based losses (Fig. 6a ). Unexpectedly, the experimental ring-down times deviate down from our theoretical predictions at f < 100 GHz. While some limitations of the measuring technique can be a contributor, we attribute most of this divergence to another extrinsic loss mechanism only recently considered in ultrathin photoexcited semiconductor plates [56] —the lateral spreading of pump-generated elastic waves that propagate outward from the probe-beam spot as Lamb waves [23] (see Supplementary Note 9 ). The escape rate of these waves, as opposed to a phonon lifetime, can be a limiting factor in the experimentally-measured ring-down at lower frequencies. Given the absence of any structurally-defined lateral confinement in our films (e.g., walls or steps), the escape time is governed by the details of Lamb wave dispersion (see Supplementary Note 10 ) and scales approximately as a ratio of pump spot size, R pump , to film thickness, h , τ Lamb ~ R pump / h , which makes the runaway more pronounced for thicker films. The analytical approach developed by Photiadis et al. [56] is consistent with FEM modeling for MoS 2 films (see Lamb wave dispersion calculated using eigenfrequency analysis and ring-down time extracted from time-domain simulations in Supplementary Figs. 18 , 19 ). The estimates for the Lamb waves escape times (LWE) produced by numerical modeling are shown by green points/line in Fig. 6a and agree well with the low frequency leveling-off of our experimentally measured ring-down times. It is evident from comparing Figs. 1 c and 3a that the ring-down time measured for h-BN-based structures is significantly shorter than that exhibited by monolithic MoS 2 films. 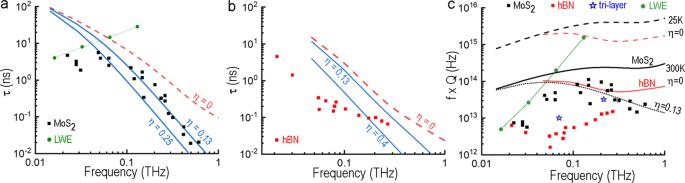Fig. 6: Experimental and theoretical results for the lifetimes of LA phonons polarized perpendicular to the basal plane. Frequency dependence predicted for the room temperature phonon lifetimes inaMoS2andbh-BN as defined by anharmonic scattering alone (dashed curves; η = 0) and by the combination of anharmonic scattering with surface losses (solid curves; η > 0) for two values of rms surface roughness (η) in nanometers. Values extracted from experimentally measured cavity ring-down times are shown by the black (a) and red (b) square points. The green points inaandcshow the FEM-calculated time for Lamb waves escape LWE (see Supplementary Note9for details).cComparison of calculated and measuredf×Qproduct as a function of frequency. The black lines showf×Qvalues calculated for MoS2cavities and the red lines correspond to h-BN structures at the labeled temperatures and η. Experimental data for cavities studied in the present work are given by the square and star symbols as labeled. The tri-layer data points represent the MoS2/h-BN/MoS2heterostructure (see Fig.4). Figure 6b shows that the phonon lifetimes in h-BN (extracted from Fig. 3b and additional h-BN/MoS 2 cavities) is consistently lower than the theoretical limit defined by phonon–phonon scattering. The dashed line in Fig. 6b is for anharmonic phonon scattering alone ( η = 0) while two solid curves show the cumulative effects of phonon–phonon as well as boundary scattering. Comparison with the experimental data shows that even the upper-bound value for h-BN surface roughness reported in the literature η = 0.1–0.4 [57] , [58] does not fully account for the extra dissipation in our devices. The presence of the h-BN/MoS 2 interface cannot explain the extra dissipation since the ring-down times from our tri-layer structure MoS 2 /h-BN/MoS 2 (which contains two identical interfaces with a very thin h-BN layer) is actually longer than the decay in the h-BN/MoS 2 bilayer with a single interface (Fig. 6c , blue stars). This discrepancy implies the presence of an additional dissipation mechanism, possibly related to inter-mode coupling or material quality. We anticipate that future low temperature measurements will provide insights into various loss mechanisms in h-BN. Finally, to gain a broader picture of how these results project the ultimate performance of 2D material-based acoustic cavities, we employ f × Q products as a figure of merit. Figure 6c compares experimental data with the f × Q values calculated for bulk MoS 2 and h-BN at two different temperatures. For anharmonicity-limited systems the predicted f × Q product increases slightly with frequency (in a qualitative agreement with the Landau–Rumer model [55] ), and for a given material represents the highest achievable performance for an acoustic cavity. With the boundary scattering term included for MoS 2 (η = 0.13) the f × Q product decreases with increasing frequency (dotted line Fig. 6c ), and fits our experimental f × Q values for MoS 2 (black squares Fig. 6c ). The order of magnitude increase in f × Q projected at low temperature is highly desirable, but will only become attainable if boundary scattering can be mitigated (see for example ref. [21] ). The presence of a “goldilocks zone” centered near f ≈ 100–200 GHz, where currently available materials and fabrication techniques yield the highest f × Q products, is an important takeaway from Fig. 6c . Being flanked by the dominance of lateral spreading of elastic waves at low frequency (green points/line) and by surface scattering at higher frequencies (black dotted line), the f × Q product at the 100–200 GHz range exceeds that required for ground state laser cooling ( f × Q = 6 × 10 12 ) by more than order of magnitude. Data from the tri-layer cavity in Fig. 4 (blue stars in Fig. 6c ) offers an example of how a relatively lossy material (h-BN) can be added judiciously to the acoustic device to expand functionality, while maintaining high overall cavity performance (see f × Q ≈ 3 × 10 13 for the 200 GHz mode of the tri-layer). We view this approach as a path toward integrated optomechanical systems where the cavity couples high-frequency elastic waves to embedded quantum systems (e.g., optical emitters in h-BN), while the acoustic interaction with the quantum system can be further tuned using advanced methods of laser cooling [59] or coherent phonon manipulation (e.g., refs. [60] , [61] , [62] ). In summary, we have shown how heterogeneities within high-quality 2D material structures extend the functionality of acoustic cavities operating in the GHz to THz frequency range. We demonstrated differential readout for adjacent MoS 2 cavities detuned by a monolayer step, as well as a frequency comb generator in a heterostructured h-BN/MoS 2 cavity. By employing MoS 2 as a thin transducer for h-BN, we successfully extracted the longitudinal phonon lifetimes for optically transparent h-BN. Strain engineering within tri-layer MoS 2 /h-BN/MoS 2 laminar structures resulted in strongly coupled acoustic cavities with coupling strengths of Γ ≈ 47 GHz. Our first-principles theoretical analysis provides a benchmark for the highest attainable, material-limited performance for 2D acoustic cavities at different temperatures. We find that the currently available 2D material quality and fabrication techniques can produce acoustic devices that operate within a factor of three of their fundamental anharmonic limit at RT, where we measure f × Q products in excess of 1 × 10 14 in vicinity of 100–200 GHz frequency range. We anticipate that by extending the palette of 2D materials and by invoking different types of heterogeneities within 2D acoustic cavities, numerous acoustic devices will become available for advanced phonon-based sensing and signal processing. Sample fabrication In order to mitigate extrinsic contributions to the acoustic losses, we fabricated 2D material structures with minimal exposure to wet chemistry agents. To fabricate samples, we first lithographically patterned and etched wells and trenches into a Si or SiO 2 /Si substrate (e.g., Fig. 1a , well diameter: 1–10 μm; well depth: 250–425 nm). Then a Ti (5 nm)/Au (40 nm) film was evaporated on the surface, which served two purposes: (i) facilitating the exfoliation of large-area samples (e.g., ref. [63] ) and (ii) to enhance the optical cavity formed between the bottom of the wells and the suspended films. Bulk MoS 2 crystals were directly exfoliated onto these substrates, leaving behind suspended flakes ranging in thickness from monolayer to bulk (see Supplementary Fig. 1 ). Measurements were performed on flakes ranging in thickness from 2.5 nm (4 L) up to 60 nm. Heterostructures (h-BN/MoS 2 and MoS 2 /h-BN/MoS 2 ) were fabricated using a PPC/PDMS stamping technique [20] where h-BN and MoS 2 films were exfoliated onto different SiO 2 substrates. The PPC/PDMS stamp was then used to sequentially pick up the predetermined layers. Afterwards the heterostructure stacks were thermally released on the well-etched substrate described above. To determine film thicknesses for MoS 2 flakes under ten layers, we use a combination of optical microscopy and Raman spectroscopy (e.g., peak positions of the interlayer breathing and shear modes of MoS 2 [64] , see Supplementary Fig. 2 ). For MoS 2 films >10 layers and for all h-BN layers we used atomic force microscopy (AFM) to measure film thickness. Pump-probe measurements An ultrafast optical pump-probe setup with micrometer-scale spatial resolution was used to study longitudinal vibrations in both MoS 2 and MoS 2 /h-BN suspended films. Two femtosecond Ti:Sapphire lasers with repetition rate ~960 MHz provided pump (750 nm wavelength, 3–10 mW power) and probe (830 nm, ≤1 mW) pulses with variable time delay governed by asynchronous optical sampling (ASOPS) [65] , [66] . The detuning between the pump and probe repetition rate was set at 2.5 kHz. Both beams were focused using 50× objective lens and independently positioned with respect to structures of interest. The same objective also provided optical imaging of the sample and was used to collect the reflected probe light. In order to facilitate optical readout, the wells in the substrate were pre-etched to a depth that approximately equals one-half the wavelength of the probe beam (λ probe ~830 nm), which forms an optical cavity between the suspended flake and bottom mirror. This configuration in combination with a high repetition rate allows us to use relatively low pulse energy in order to provide acceptable signal-to-noise ratio while mitigating overheating and ensuring linear response of the mechanical structure. Typical acquisition mode included 50,000 sweeps averaged over accumulation time of 20 s. All the measurements were done at RT in ambient conditions. Phonon lifetime calculations For first-principles calculations, the strength of each scattering is determined by matrix elements built from third-order anharmonic perturbations, frequencies, and eigenvectors of the phonons [51] , [53] , [67] derived from DFT. Phonon scattering due to point defects, such as isotopic variation, is negligible for the frequency range considered here, particularly around RT. This method has been found to give good agreement with measured data in a wide range of bulk materials for phonon dispersions [68] , [69] , [70] and for thermal conductivities [67] , [71] , [72] , where the latter are governed by phonon scattering. Details are given in the Supplementary Notes 7 , 8 .